Origin and cross-species transmission of bat coronaviruses in China Bats are presumed reservoirs of diverse coronaviruses (CoVs) including progenitors of Severe Acute Respiratory Syndrome (SARS)-CoV and SARS-CoV-2, the causative agent of COVID-19. However, the evolution and diversification of these coronaviruses remains poorly understood. Here we use a Bayesian statistical framework and a large sequence data set from bat-CoVs (including 630 novel CoV sequences) in China to study their macroevolution, cross-species transmission and dispersal. We find that host-switching occurs more frequently and across more distantly related host taxa in alpha- than beta-CoVs, and is more highly constrained by phylogenetic distance for beta-CoVs. We show that inter-family and -genus switching is most common in Rhinolophidae and the genus Rhinolophus . Our analyses identify the host taxa and geographic regions that define hotspots of CoV evolutionary diversity in China that could help target bat-CoV discovery for proactive zoonotic disease surveillance. Finally, we present a phylogenetic analysis suggesting a likely origin for SARS-CoV-2 in Rhinolophus spp. bats. Coronaviruses (CoVs) are RNA viruses causing respiratory and enteric diseases with varying pathogenicity in humans and animals. All CoVs known to infect humans are zoonotic, or of animal origin, with many thought to originate in bat hosts [1] , [2] . Due to their large genome size (the largest non-segmented RNA viral genome), frequent recombination, and high genomic plasticity, CoVs are prone to cross-species transmission and are able to rapidly adapt to new hosts [1] , [3] . This phenomenon is thought to have led to the emergence of a number of CoVs affecting livestock and human health [4] , [5] , [6] , [7] , [8] , [9] . Severe Acute Respiratory Syndrome (SARS)-CoV was reported first in humans in Guangdong province, southern China, in 2002 and caused fatal respiratory infections in close to 800 people worldwide [10] , [11] , [12] . Subsequent investigations identified horseshoe bats (genus Rhinolophus ) as the natural reservoirs of SARS-related CoVs and the likely origin of SARS-CoV [13] , [14] , [15] , [16] . In 2016, Swine Acute Diarrhea Syndrome (SADS)-CoV caused the death of over 25,000 pigs in farms within Guangdong province [17] . This virus appears to have originated within Rhinolophus spp. bats, and belongs to the HKU2-CoV clade previously detected in bats in the region [17] , [18] , [19] . In 2019, a novel CoV (SARS-CoV-2) causing respiratory illness (COVID-19) was first reported in Wuhan, Hubei province, China. This emerging human virus is closely related to SARS-CoV, and also appears to have originated in horseshoe bats [20] , [21] —with its full genome 96% similar to a viral sequence reported from Rhinolophus affinis [20] . Closely related sequences were also identified in Malayan pangolins [22] , [23] . A growing body of research has identified bats as the evolutionary sources of SARS—and Middle East Respiratory Syndrome (MERS)—CoVs [13] , [14] , [24] , [25] , [26] , and as the source of progenitors for the human CoVs, NL63 and 229E [27] , [28] . The emergence of SARS-CoV-2 further underscores the importance of bat-origin CoVs to global health, and understanding their origin and cross-species transmission is a high priority for pandemic preparedness [20] , [29] . Bats harbor the largest diversity of CoVs among mammals, and two CoV genera, α- and β-CoVs have been widely detected in bats from most regions of the world [30] , [31] . Bat-CoV diversity seems to be correlated with host taxonomic diversity globally, with the highest CoV diversity being found in areas with the highest bat species richness [32] . Host switching of viruses over evolutionary time is an important mechanism driving the evolution of bat-CoVs in nature and appears to vary geographically [32] , [33] . However, detailed analyses of host switching have been hampered by incomplete or opportunistic sampling, typically with relatively low numbers of viral sequences from any given region [34] . China has a rich bat fauna, with more than 100 described bat species and several endemic species representing both the Palearctic and Indo-Malay regions [35] . Its situation at the crossroads of two zoogeographic regions heightens China’s potential to harbor a unique and distinctive CoV diversity. Since the emergence of SARS-CoV in 2002, China has been the focus of an intense viral surveillance and a large number of diverse bat-CoVs have been discovered in the region [36] , [37] , [38] , [39] , [40] , [41] , [42] , [43] , [44] . However, the macroevolution of CoVs in their bat hosts in China and their cross-species transmission dynamics remain poorly understood. In this study, we analyze an extensive field-collected dataset of bat-CoV sequences from across China. We use a phylogeographic Bayesian statistical framework to reconstruct virus transmission history between different bat host species and virus spatial spread over evolutionary time. Our objectives are to compare the macroevolutionary patterns of α- and β-CoVs and identify the hosts and geographical regions that act as centers of evolutionary diversification for bat-CoVs in China. These analyses aim to improve our understanding of how CoVs evolve, diversify, circulate among, and transmit between bat families and genera to help identify bat hosts and regions where the risk of CoV spillover is the highest. Taxonomic and geographic sampling We generated 630 partial sequences (440 nt) of the RNA-dependent RNA polymerase ( RdRp ) gene from bat rectal swabs collected in China and added 608 bat-CoV and 8 pangolin-CoV sequences from China available in GenBank or GISAID to our datasets (list of GenBank and GISAID accession numbers available in Supplementary Note 1 ). For each CoV genus, two datasets were created: one including all bat-CoV sequences with known host (host dataset) and one including all bat-CoV sequences with known sampling location at the province level (geographic dataset). To create a geographically discrete partitioning scheme that was more ecologically relevant than administrative borders for our phylogeographic reconstructions, we defined six zoogeographic regions within China by clustering provinces with similar mammalian diversity using hierarchical clustering [45] (see “Methods”): South western region (SW), Northern region (NO), Central northern region (CN), Central region (CE), Southern region (SO), and Hainan island (HI) (Fig. 1 and Supplementary Fig. 1 ). Fig. 1: Geographic sampling. Pie chart ( a ) showing the number of sequences of each CoV genus (α-CoVs and β-CoVs) available for each zoogeographic region and map of China provinces ( b ) showing the number of RdRp sequences available for each province, in bold gray for α-CoVs and black for β-CoVs. Province colors correspond to the zoogeographic region to which they belong: NO Northern region, CN Central northern region, SW South western region, CE Central region, SO Southern region, HI Hainan island. The three β-CoV sequences from HI were included in the SO region. Provinces colored in gray are those where CoV sequences are not available. 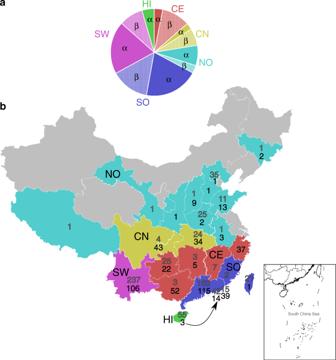Fig. 1: Geographic sampling. Pie chart (a) showing the number of sequences of each CoV genus (α-CoVs and β-CoVs) available for each zoogeographic region and map of China provinces (b) showing the number ofRdRpsequences available for each province, in bold gray for α-CoVs and black for β-CoVs. Province colors correspond to the zoogeographic region to which they belong: NO Northern region, CN Central northern region, SW South western region, CE Central region, SO Southern region, HI Hainan island. The three β-CoV sequences from HI were included in the SO region. Provinces colored in gray are those where CoV sequences are not available. Full size image Our host datasets included 701 α-CoV sequences (353 new sequences, including 102 new SADSr-CoV sequences ( Rhinacovirus )) from 41 bat species (14 genera, five families) and 528 β-CoV sequences (273 new sequences, including 97 new SARSr-CoV sequences ( Sarbecovirus )) from 31 bat species (15 genera, four families) (Supplementary Table 1 ). Our geographic datasets included 677 α-CoV sequences from six zoogeographic regions (22 provinces) and 503 β-CoV sequences from five zoogeographic regions (21 provinces) (Fig. 1 ). As some regions or hosts were overrepresented in our datasets, we also created and ran our analyses using a more uniform subset of our sequence data that included ~30 randomly selected sequences per host family or region to mitigate sampling and surveillance intensity bias. Ancestral hosts and cross-species transmission We used a Bayesian discrete phylogeographic approach implemented in BEAST [46] to reconstruct the ancestral host of each node in the phylogenetic tree using bat host family as a discrete character state. The phylogenetic reconstructions for α-CoVs in China suggest an evolutionary origin within rhinolophid and vespertilionid bats (Fig. 2a ). The first α-CoV lineage to diverge historically corresponds to the subgenus Rhinacovirus (L1), originating within rhinolophid bats, and includes sequences related to HKU2-CoV and SADS-CoV (Supplementary Fig. 2 ). Then, several lineages, labeled L2–L7, emerged from vespertilionid bats (Fig. 2a ). The subgenus Decacovirus (L2) includes sequences mostly associated with the Rhinolophidae and Hipposideridae and related to HKU10-CoV (Supplementary Fig. 3 ), while the subgenera Myotacovirus (L3) and Pedacovirus (L5), as well as an unidentified lineage (L4), include CoVs mainly from vespertilionid bats and related to HKU6-CoV, HKU10-CoV, and 512-CoV (Supplementary Figs. 4 and 5 ). Finally, a well-supported node comprises the subgenera Nyctacovirus (L6) from vespertilionid bats and Minunacovirus (L7) from miniopterid bats, and includes HKU7-CoV, HKU8-CoV, 1A-CoV, and 1B-CoV (Supplementary Fig. 6 ). These seven α-CoV lineages are mostly associated with a single host family, but each also included several sequences identified from other bat families (Fig. 2a , Supplementary Figs. 2 – 6 , and Supplementary Table 1 ), suggesting that frequent cross-species transmission events have occurred among bats. Ancestral host reconstructions based on the random data subset, to normalize sampling effort, gave very similar results, with rhinolophids and vespertilionids being the most likely ancestral hosts of most α-CoV lineages too (Supplementary Fig. 7A ). However, the topology of the tree based on the random subset was slightly different as the lineage L5 was paraphyletic. Fig. 2: Phylogenetic trees and ancestral host reconstructions. α-CoV ( a ) and β-CoV ( b ) maximum clade credibility annotated trees using complete datasets of RdRp sequences and bat host family as discrete character state. Pie charts located at the root and close to the deepest nodes show the state posterior probabilities for each bat family. Branch colors correspond to the inferred ancestral family with the highest probability. Branch lengths are scaled according to relative time units (clock rate = 1.0). Well-supported nodes (posterior probability > 0.95) are indicated with a black dot. The ICTV approved CoV subgenera were highlighted: Rhinacovirus (L1), Decacovirus (L2), Myotacovirus (L3), Pedacovirus (L5), Nyctacovirus (L6), Minunacovirus (L7), and an unidentified lineage (L4) for α-CoVs; and Merbecovirus (Lineage C), Nobecovirus (lineage D), Hibecovirus (lineage E), and Sarbecovirus (Lineage B) for β-CoVs. Full size image Chinese β-CoVs likely originated from vespertilionid and rhinolophid bats (Fig. 2b ). The maximum clade credibility (MCC) tree was clearly structured into four main lineages: Merbecovirus (lineage C), including MERS-related (MERSr-) CoVs, HKU4-CoV, and HKU5-CoV, and strictly restricted to vespertilionid bats (Supplementary Fig. 8 ); Nobecovirus (lineage D), originating from pteropodid bats and corresponding to HKU9-CoV (Supplementary Fig. 9 ); Hibecovirus (lineage E), comprising sequences isolated in hipposiderid bats (Supplementary Fig. 10 ) and Sarbecovirus (lineage B), including sequences related to HKU3- and SARS-related (SARSr-) CoVs originating in rhinolophid bats (Supplementary Fig. 11 ). We show that SARS-CoV-2 forms a divergent clade within Sarbecovirus and is most closely related to viruses sampled from Rhinolophus malayanus and R. affinis and from Malayan pangolins ( Manis javanica ) (Fig. 3 ). Similar tree topology and ancestral host inference were obtained with the random subset (Supplementary Fig. 7B ). Fig. 3: Phylogenetic relationships within the Sarbecovirus subgenus (β-CoVs). Maximum clade credibility tree ( a ) including 202 RdRp sequences from the Sarbecovirus subgenus isolated in bats, two sequences of SARS-CoV-2, and one sequence of SARS-CoV isolated in humans and eight sequences isolated in Malayan pangolins ( Manis javanica ). Well-supported nodes (posterior probability > 0.95) are indicated with a black dot. Tip colors correspond to the host genus; SARS-CoV-2 sequences and SARS-CoV sequence are highlighted in gray and black, respectively. Median-joining network ( b ) including 202 RdRp sequences from the Sarbecovirus lineage isolated in bats, two sequences of SARS-CoV-2, and one sequence of SARS-CoV isolated in humans and eight sequences isolated in Malayan pangolins ( Manis javanica ). Colored circles correspond to distinct CoV sequences, and circle size is proportional to the number of identical sequences in the dataset. Small black circles represent median vectors (ancestral or unsampled intermediate sequences). Branch length is proportional to the number of mutational steps between haplotypes. Full size image We used a Bayesian stochastic search variable selection (BSSVS) procedure [47] to identify viral host switches (transmission over evolutionary time) between bat families and genera that occurred along the branches of the MCC annotated tree and calculated Bayesian factor (BF) to estimate the significance of these switches (Fig. 4 ). We identified nine highly supported (BF > 10) inter-family host switches for α-CoVs and three for β-CoVs (Fig. 4a, b ). These results are robust over a range of sample sizes, with seven of these nine switches for α-CoVs and the exact same three host switches for β-CoVs having strong BF support (BF > 10) when analyzing our random subset (Supplementary Tables 2 and 3 ). To quantify the magnitude of these host switches, we estimated the number of host-switching events (Markov jumps) [48] , [49] along the significant inter-family switches (Fig. 4c, d ) and estimated the rate of inter-family host-switching events per unit of time for each CoV genus. The rate of inter-family host-switching events was five times higher in the evolutionary history of α-CoVs (0.010 host switches/unit time) than β-CoVs (0.002 host switches/unit time) in China. For α-CoVs, host-switching events from the Rhinolophidae and the Miniopteridae were greater than from other bat families, while rhinolophids were the highest donor family for β-CoVs. The Rhinolophidae and the Vespertilionidae for α-CoVs and the Hipposideridae for β-CoVs received the highest numbers of switching events (Fig. 4c, d ). When using the random dataset, similar results were obtained for β-CoVs, while rhinolophids were the highest donor family for α-CoVs (Supplementary Tables 4 and 5 ). Fig. 4: Inter-family host switches. Strongly supported host switches between bat families for α-CoVs ( a ) and β-CoVs ( b ). Arrows indicate the direction of the switch; arrow thickness is proportional to the switch significance level, only host switches supported by strong Bayes factor (BF) > 10 are shown. Histograms of total number of host-switching events (state changes counts using Markov jumps) from/to each bat family along the significant inter-family switches for α-CoVs ( c ) and β-CoVs ( d ). Full size image At the genus level, we identified 20 highly supported inter-genus host switches for α-CoVs, 17 of them were also highly significant using the random subset (Fig. 5a and Supplementary Table 6 ). Sixteen highly supported inter-genus switches were identified for β-CoVs (Fig. 5b ). Similar results were obtained for the random β-CoV subset (Supplementary Table 7 ). 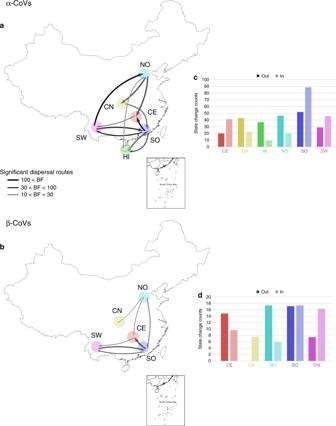Fig. 6: CoV spatiotemporal dispersal in China. Strongly supported dispersal routes (Bayes factor, BF > 10) over recent evolutionary history among China zoogeographic regions for α-CoVs (a) and β-CoVs (b). Arrows indicate the direction of the dispersal route; arrow thickness is proportional to the dispersal route significance level. Darker arrow colors indicate older dispersal events. Histograms of total number of dispersal events (Markov jumps) from/to each region along the significant dispersal routes for α-CoVs (c) and β-CoVs (d). NO Northern region, CN Central northern region, SW South western region, CE Central region, SO Southern region, HI Hainan island. Most of the significant cross-genus CoV switches for α-CoVs, 15 of 20 (75%), were between genera in different bat families, while this proportion was only 6 of 16 (37.5%) for β-CoVs. The estimated rate of inter-genus host-switching events (Markov jumps) was similar for α-CoVs (0.014 host switches/unit time) and β-CoVs (0.014 host switches/unit time). For α-CoVs, Rhinolophus and Miniopterus were the greatest donor genera and Rhinolophus was the greatest receiver (Supplementary Table 8 ). 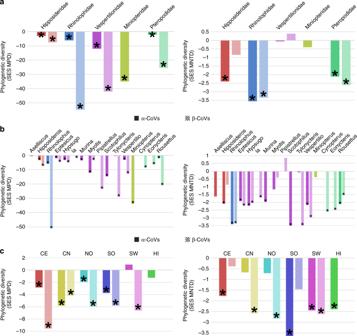Fig. 7: Phylogenetic diversity. Metrics of CoV phylogenetic diversity within each bat family (a), genus (b), and zoogeographic regions (c): standardized effect size of mean phylogenetic distance (SES MPD), on the left panels; and standardized effect size of mean nearest taxon distance (SES MNTD), on the right panels. One-tailedpvalues (quantiles) were calculated after randomly reshuffling tip labels 1000 times along the entire phylogeny. Values departing significantly from the null model (pvalue < 0.05) are indicated with an asterisk, all exactpvalues are available in Supplementary Tables14–27. NO Northern region, CN Central northern region, SW South western region, CE Central region, SO Southern region, HI Hainan island. For β-CoVs, Rousettus was the greatest donor and Eonycteris the greatest receiver genus (Supplementary Table 9 ). Fig. 5: Inter-genus host switches. 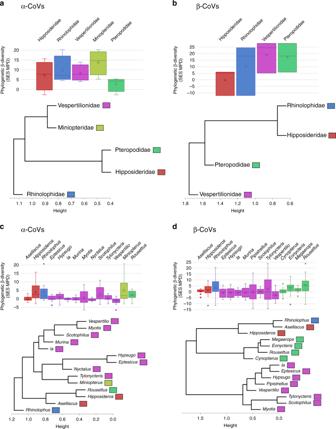Fig. 8: Phylogenetic diversity. Standardized effect size of mean phylogenetic distance (SES MPD) and phylogenetic ordination among bat host families (a,b) and genera (c,d) for α- and β-CoVs. Boxplots for each host family and genus show the mean (cross), median (dark line within the box), interquartile range (box), 95% confidence interval (whisker bars), and outliers (dots), calculated from all pairwise comparisons between bat families (n= 10 for α-CoVs andn= 6 for β-CoVs) and genera (n= 91 for α-CoVs andn= 105 for β-CoVs). Strongly supported host switches between bat genera for α-CoVs ( a ) and β-CoVs ( b ) and their significance level (Bayes factor, BF). 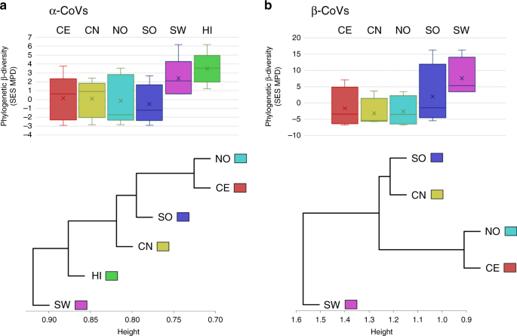Fig. 9: Phylogenetic diversity. Standardized effect size of mean phylogenetic distance (SES MPD) and phylogenetic ordination among zoogeographic regions for α-CoVs (a) and β-CoVs (b). Boxplots for each region show the mean (cross), median (dark line within the box), interquartile range (box), 95% confidence interval (whisker bars), and outliers (dots), calculated from all pairwise comparisons between regions (n= 15 for α-CoVs andn= 10 for β-CoVs). NO Northern region, CN Central northern region, SW South western region, CE Central region, SO Southern region, HI Hainan island. Only host switches supported by strong BF values >10 are shown. Line thickness is proportional to the switch significance level. Red lines correspond to host switches among bat genera belonging to different families, and black lines correspond to host switches among bat genera from the same family. Arrows indicate the direction of the switch. Genus names are colored according to the family they belong to using the same colors as in Figs. 2 and 3 . Full size image CoV spatiotemporal dispersal in China We used our Bayesian discrete phylogeographic model with zoogeographic regions as character states to reconstruct the spatiotemporal dynamics of CoV dispersal in China. Eleven and seven highly significant (BF > 10) dispersal routes within China were identified for α- and β-CoVs, respectively (Fig. 6 ). Seven and five of these dispersal routes, respectively, remained significant when using our random subsets (Supplementary Tables 10 and 11 ). The Rhinacovirus lineage (L1) that includes HKU2-CoV and SADS-CoV likely originated in the SO region, while all other α-CoV lineages historically arose in SW China and spread to other regions before several dispersal events from SO and NO in all directions (Fig. 6a and Supplementary Fig. 12 ). A roughly similar pattern of α-CoV dispersal was obtained using the random subset (Supplementary Tables 10 and 12 ). Fig. 6: CoV spatiotemporal dispersal in China. Strongly supported dispersal routes (Bayes factor, BF > 10) over recent evolutionary history among China zoogeographic regions for α-CoVs ( a ) and β-CoVs ( b ). Arrows indicate the direction of the dispersal route; arrow thickness is proportional to the dispersal route significance level. Darker arrow colors indicate older dispersal events. Histograms of total number of dispersal events (Markov jumps) from/to each region along the significant dispersal routes for α-CoVs ( c ) and β-CoVs ( d ). NO Northern region, CN Central northern region, SW South western region, CE Central region, SO Southern region, HI Hainan island. Full size image The oldest inferred dispersal movements for β-CoVs occurred among the SO and SW regions (Fig. 6b ). The SO region was the likely origin of Merbecovirus (lineage C, including HKU4-CoV and HKU5-CoV) and Sarbecovirus subgenera (lineage B, including HKU3-CoV and SARSr-CoV), while the Nobecovirus (lineage D, including HKU9-CoV) and Hibecovirus (lineage E) subgenera originated in SW China (Supplementary Fig. 12 ). Then, several dispersal movements likely originated from SO and CE (Fig. 6b ). More recent southward dispersal from NO was observed. Similar spatiotemporal dispersal patterns were observed using the random subset of β-CoVs (Supplementary Tables 11 and 13 ). The estimated rate of migration events per unit of time along these significant dispersal routes was more than two times higher for α-CoVs (0.026 host switches/unit time) than β-CoVs (0.011 host switches/unit time), and SO was the region involved in the greatest total number of migration events for both α- and β-CoVs. SO had the highest number of outbound and inbound migration events for α-CoVs (Fig. 6c and Supplementary Table 12 ). For β-CoVs, the highest number of outbound migration events was estimated to be from NO and SO, while SO and SW had the highest numbers of inbound migration events (Fig. 6d and Supplementary Table 13 ). Phylogenetic diversity In order to identify the hotspots of CoV phylogenetic diversity in China and evaluate phylogenetic clustering of CoVs, we calculated the mean phylogenetic distance (MPD) and the mean nearest taxon distance (MNTD) statistics [50] and their standardized effect size (SES). We found significant and negative SES MPD values, indicating significant phylogenetic clustering, within all bat families and genera for both α- and β-CoVs, except within the Aselliscus and Tylonycteris for α-CoVs (Fig. 7a, b ). Negative and mostly significant SES MNTD values, reflecting phylogenetic structure closer to the tips, were also observed within most bat families and genera for α- and β-CoVs, but we found nonsignificant positive SES MNTD value for vespertilionid bats, and particularly for those in the Pipistrellus genus, for β-CoVs (Fig. 7a, b ). In general, we observed lower phylogenetic diversity for β-CoVs than α-CoVs within all bat families and most genera when looking at SES MPD, but the difference in the level of diversity between α- and β-CoVs is less important when looking at SES MNTD (Fig. 7 ). These results suggest stronger basal clustering (reflected by larger SES MPD values) for β-CoVs than α-CoVs, indicating stronger host structuring effect and phylogenetic conservatism for β-CoVs. Very similar results were obtained with the random subsets for both α- and β-CoVs (Supplementary Tables 14 – 21 ). Fig. 7: Phylogenetic diversity. Metrics of CoV phylogenetic diversity within each bat family ( a ), genus ( b ), and zoogeographic regions ( c ): standardized effect size of mean phylogenetic distance (SES MPD), on the left panels; and standardized effect size of mean nearest taxon distance (SES MNTD), on the right panels. One-tailed p values (quantiles) were calculated after randomly reshuffling tip labels 1000 times along the entire phylogeny. Values departing significantly from the null model ( p value < 0.05) are indicated with an asterisk, all exact p values are available in Supplementary Tables 14 – 27 . NO Northern region, CN Central northern region, SW South western region, CE Central region, SO Southern region, HI Hainan island. Full size image We found negative and mostly significant values of MPD and MNTD (Fig. 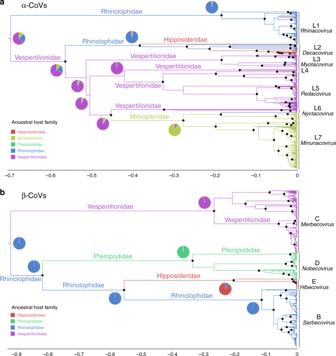7c and Supplementary Tables 22 – 25 ) indicating significant phylogenetic clustering of CoV lineages in bat communities within the same zoogeographic region. However, SES MPD values for α-CoVs in SW were positive (significant for the random subset), indicating a greater evolutionary diversity of CoVs in that region than others (Fig. 7 and Supplementary Tables 22 – 25 ). We used a linear regression analysis to assess the relationship between CoV phylogenetic diversity and bat species richness in China and determine if bat richness is a significant predictor of bat-CoV diversity and evolution. Fig. 2: Phylogenetic trees and ancestral host reconstructions. α-CoV (a) and β-CoV (b) maximum clade credibility annotated trees using complete datasets ofRdRpsequences and bat host family as discrete character state. Pie charts located at the root and close to the deepest nodes show the state posterior probabilities for each bat family. Branch colors correspond to the inferred ancestral family with the highest probability. Branch lengths are scaled according to relative time units (clock rate = 1.0). Well-supported nodes (posterior probability > 0.95) are indicated with a black dot. The ICTV approved CoV subgenera were highlighted:Rhinacovirus(L1),Decacovirus(L2),Myotacovirus(L3),Pedacovirus(L5),Nyctacovirus(L6),Minunacovirus(L7), and an unidentified lineage (L4) for α-CoVs; andMerbecovirus(Lineage C),Nobecovirus(lineage D),Hibecovirus(lineage E), andSarbecovirus(Lineage B) for β-CoVs. α-CoV phylogenetic diversity (MPD) was not significantly correlated to total bat species richness or sampled bat species richness in zoogeographic regions or provinces (Supplementary Table 26 ). Nonsignificant correlations between bat species richness and β-CoV phylogenetic diversity were also observed at the zoogeographic region level (Supplementary Table 27 ). However, a significant correlation was observed between sampled bat species richness and β-CoV phylogenetic diversity at the province level (Supplementary Table 27 ). Similar results were obtained when using the random subsets (Supplementary Tables 26 and 27 ). These findings suggest that bat host diversity is not the main driver of CoV diversity in China and that other ecological or biogeographic factors may influence this diversity. We observed higher CoV diversity than expected in several southern or central provinces (Hainan, Guangxi, Hunan) given their underlying total or sampled bat diversity (Supplementary Figs. 13 and 14 ). We also assessed patterns of CoV phylogenetic turnover/differentiation among Chinese zoogeographic regions and bat host families by measuring the inter-region and inter-host values of MPD (equivalent to a measure of phylogenetic β-diversity) and their SES. We found positive inter-family SES MPD values, except between Pteropodidae and Hipposideridae for α-CoVs and between Rhinolophidae and Hipposideridae for β-CoVs (Fig. 8a, b and Supplementary Tables 28 and 29 ), suggesting higher phylogenetic differentiation of CoVs among most bat families than among random communities. Our phylo-ordination based on inter-family MPD values indicated that α-CoVs from vespertilionids and miniopterids, and from hipposiderids and pteropodids, as well as β-CoVs from rhinolophids and hipposiderids, were phylogenetically closely related (Fig. 8a, b ). We also observed strong phylogenetic turnover between α-CoV strains from rhinolophids and from miniopterids and all other bat families, and between β-CoV strains from vespertilionids and all other bat families (Supplementary Tables 28 and 29 ). Phylo-ordination among bat genera based on inter-genus MPD confirmed these results and indicated that CoV strains from genera belonging to the same bat family were mostly more closely related to each other than to genera from other families (Fig. 8c, d and Supplementary Tables 30 and 31 ). Fig. 8: Phylogenetic diversity. Standardized effect size of mean phylogenetic distance (SES MPD) and phylogenetic ordination among bat host families ( a , b ) and genera ( c , d ) for α- and β-CoVs. Boxplots for each host family and genus show the mean (cross), median (dark line within the box), interquartile range (box), 95% confidence interval (whisker bars), and outliers (dots), calculated from all pairwise comparisons between bat families ( n = 10 for α-CoVs and n = 6 for β-CoVs) and genera ( n = 91 for α-CoVs and n = 105 for β-CoVs). Full size image We observed high and positive inter-region SES MPD values between SW/HI and all other regions, suggesting that these two regions host higher endemic diversity (Fig. 9 and Supplementary Tables 32 and 31 ). Negative inter-region SES MPD values suggested that the phylogenetic turnover among other regions was less important than expected among random communities. Our phylo-ordination among zoogeographic regions also reflected the high phylogenetic turnover and deep evolutionary distinctiveness of both α- and β-CoVs from SW and HI regions (Fig. 9 and Supplementary Tables 32 and 33 ). Similar results were obtained using the random subset (Supplementary Tables 32 and 33 ). Fig. 9: Phylogenetic diversity. Standardized effect size of mean phylogenetic distance (SES MPD) and phylogenetic ordination among zoogeographic regions for α-CoVs ( a ) and β-CoVs ( b ). Boxplots for each region show the mean (cross), median (dark line within the box), interquartile range (box), 95% confidence interval (whisker bars), and outliers (dots), calculated from all pairwise comparisons between regions ( n = 15 for α-CoVs and n = 10 for β-CoVs). NO Northern region, CN Central northern region, SW South western region, CE Central region, SO Southern region, HI Hainan island. Full size image Mantel tests Mantel tests revealed a positive and significant correlation between CoV genetic differentiation ( F ST ) and geographic distance matrices, both with and without provinces, including fewer than four viral sequences, for α-CoVs ( r = 0.25, p = 0.0097; r = 0.32, p = 0.0196; respectively) and β-CoVs ( r = 0.22, p = 0.0095; r = 0.23, p = 0.0336; respectively). We also detected a positive and highly significant correlation between CoV genetic differentiation ( F ST ) and their host phylogenetic distance matrices, both with and without genera, including fewer than four viral sequences, for β-CoVs ( r = 0.41, p = 0; r = 0.39, p = 0.0012; respectively) but not for α-CoVs ( r = −0.13, p = 0.8413; r = 0.02, p = 0.5019; respectively). Our phylogenetic analysis shows a high diversity of CoVs from bats sampled in China, with most bat genera included in this study (10/16) infected by both α- and β-CoVs. In our phylogenetic analysis that includes all known bat-CoVs from China, we found that SARS-CoV-2 is likely derived from a clade of viruses originating in horseshoe bats ( Rhinolophus spp.). The geographic location of this origin appears to be Yunnan province. However, it is important to note that: (1) our study collected and analyzed samples solely from China; (2) many sampling sites were close to the borders of Myanmar and Lao PDR; and (3) most of the bats sampled in Yunnan also occur in these countries, including R. affinis and R. malayanus , the species harboring the CoVs with highest RdRp sequence identity to SARS-CoV-2 [20] , [21] . For these reasons, we cannot rule out an origin for the clade of viruses that are progenitors of SARS-CoV-2 that is outside China, and within Myanmar, Lao PDR, Vietnam, or another Southeast Asian country. Additionally, our analysis shows that the virus RmYN02 from R. malayanus , which is characterized by the insertion of multiple amino acids at the junction site of the S1 and S2 subunits of the Spike (S) protein, belongs to the same clade as both RaTG13 and SARS-CoV-2, providing further support for the natural origin of SARS-CoV-2 in Rhinolophus spp. bats in the region [20] , [21] . Finally, while our analysis shows that the RdRp sequences of CoVs from the Malayan pangolin are closely related to SARS-CoV-2 RdRp, analysis of full genomes of these viruses suggest that these terrestrial mammals are less likely to be the origin of SARS-CoV-2 than Rhinolophus spp. bats [22] , [23] . This analysis also demonstrates that a significant amount of cross-species transmission has occurred among bat hosts over evolutionary time. Our Bayesian phylogeographic inference and analysis of host switching showed varying levels of viral connectivity among bat hosts and allowed us to identify significant host transitions that appear to have occurred during bat-CoV evolution in China. We found that bats in the family Rhinolophidae (horseshoe bats) played a key role in the evolution and cross-species transmission history of α-CoVs. The family Rhinolophidae and the genus Rhinolophus were involved in more inter-family and inter-genus highly significant host switching of α-CoVs than any other family or genus. They were the greatest receivers of α-CoV host-switching events and second greatest donors after Miniopteridae/ Miniopterus . The Rhinolophidae, together with the Hipposideridae, also played an important role in the evolution of β-CoVs, being at the origin of most inter-family host-switching events. Chinese horseshoe bats are characterized by a distinct and evolutionarily divergent α-CoV diversity, while their β-CoV diversity is similar to that found in the Hipposideridae. The Rhinolophidae comprises a single genus, Rhinolophus , and is the most speciose bat family after the Vespertilionidae in China [51] , with 20 known species, just under a third of global Rhinolophus diversity, mostly in Southern China [35] . This family likely originated in Asia [52] , [53] , but some studies suggest an African origin [54] , [55] . Rhinolophid fossils from the middle Eocene (38–47.8 Mya) have been found in China, suggesting a westward dispersal of the group from eastern Asia to Europe [56] . The ancient likely origin of the Rhinolophidae in Asia and China in particular may explain the central role they played in the evolution and diversification of bat-CoVs in this region, including SARSr-CoVs, MERS-cluster CoVs, and SADSr-CoVs, which contain important human and livestock pathogens. Horseshoe bats are known to share roosts with genera from all other bat families in this study [57] , which may also favor CoV cross-species transmission from and to rhinolophids [34] . A global meta-analysis showing higher rates of viral sharing among co-roosting cave bats supports this finding [58] . Vespertilionid and miniopterid bats (largely within the Myotis and Miniopterus genera) also appear to have been involved in several significant host switches during α-CoV evolution. However, no significant transition from vespertilionid bats was identified for β-CoVs and these bats exhibit a divergent β-CoV diversity compared to other bat families. Vespertilionid and miniopterid bats are characterized by strong basal phylogenetic clustering, but high recent CoV diversification rates, indicating a more rapid evolutionary radiation of CoVs in these bat hosts. At the genus level, similar findings were observed for the genera Myotis , Pipistrellus , and Miniopterus . A significant correlation between geographic distance and genetic differentiation of both α- and β-CoVs has been detected, even if only a relatively small proportion of the variance is explained by geographic distance. We also revealed a significant effect of host phylogeny on β-CoV evolution while it had a minimal effect on α-CoV diversity. Contrary to the α-CoV phylogeny, the basal phylogenetic structure of β-CoVs mirrored the phylogeny of their bat hosts, with a clear distinction between the Yangochiroptera, encompassing the Vespertilionidae and Miniopteridae, and the Yinpterochiroptera, which includes the megabat family Pteropodidae and the microbat families Rhinolophidae and Hipposideridae, as evidenced in recent bat phylogenies [52] , [59] . These findings suggest a profound co-macroevolutionary process between β-CoVs and their bat hosts, even if host switches also occurred throughout their evolution as our study showed. 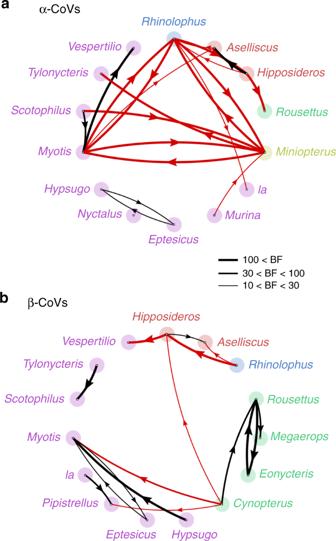The phylogenetic structure of α-CoVs, with numerous and closely related lineages identified in the Vespertilionidae and Miniopteridae, contrasts with the β-CoV macroevolutionary pattern and suggests α-CoVs have undergone an adaptive radiation in these two Yangochiroptera families. Our BSSVS procedure and Markov jump estimates revealed higher connectivity, both qualitatively and quantitatively, among bat families and genera in the α-CoV cross-species transmission history. Larger numbers of highly significant host transitions and higher rates of switching events along these pathways were inferred for α- than β-CoVs, especially at the host family level. These findings suggest that α-CoVs are able to switch hosts more frequently and between more distantly related taxa, and that phylogenetic distance among hosts represents a higher constraint on host switches for β- than α-CoVs. Fig. 5: Inter-genus host switches. Strongly supported host switches between bat genera for α-CoVs (a) and β-CoVs (b) and their significance level (Bayes factor, BF). Only host switches supported by strong BF values >10 are shown. Line thickness is proportional to the switch significance level. Red lines correspond to host switches among bat genera belonging to different families, and black lines correspond to host switches among bat genera from the same family. Arrows indicate the direction of the switch. Genus names are colored according to the family they belong to using the same colors as in Figs.2and3. This is supported by more frequent dispersal events in the evolution of α- than β-CoVs in China. 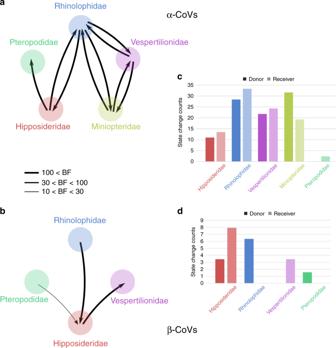Variation in the extent of host jumps between α- and β-CoVs within the same hosts in the same environment may be due to virus-specific factors, such as differences in receptor usage between α- and β-CoVs [60] , [61] , [62] . CoVs use a large diversity of receptors, and their entry into host cells is mediated by the spike protein with an ectodomain consisting of a receptor-binding subunit S1 and a membrane-fusion subunit S2 [63] . However, despite differences in the core structure of their S1 receptor-binding domains, several α- and β-CoV species are able to recognize and bind to the same host receptors [64] . Other factors such as mutation rate, recombination potential, or replication rate might also be involved in differences in host-switching potential between α- and β-CoVs. A better understanding of receptor usage and other biological characteristics of these bat-CoVs may help predict their cross-species transmission and zoonotic potential. Fig. 4: Inter-family host switches. Strongly supported host switches between bat families for α-CoVs (a) and β-CoVs (b). Arrows indicate the direction of the switch; arrow thickness is proportional to the switch significance level, only host switches supported by strong Bayes factor (BF) > 10 are shown. Histograms of total number of host-switching events (state changes counts using Markov jumps) from/to each bat family along the significant inter-family switches for α-CoVs (c) and β-CoVs (d). We also found that some bat genera were infected by a single CoV genus: Miniopterus (Miniopteridae) and Murina (Vespertilionidae) carried only α-CoVs, while Cynopterus , Eonycteris , Megaerops (Pteropodidae), and Pipistrellus (Vespertilionidae) hosted only β-CoVs. This was found despite using the same conserved pan-CoV polymerase chain reaction (PCR) assays for all specimens screened and it cannot be explained by differences in sampling effort for these genera (Supplementary Table 1 ): for example, >250 α-CoV sequences but no β-CoV sequences were discovered in Miniopterus bats in China during our recent fieldwork. These migratory bats, which seem to have played a key role in the evolution of α-CoVs, share roosts with several other bat genera hosting β-CoVs in China [57] , suggesting high likelihood of being exposed to β-CoVs. Biological or ecological properties of miniopterid bats may explain this observation and clearly warrant further investigation. Our Bayesian ancestral reconstructions revealed the importance of South western and Southern China as centers of diversification for both α- and β-CoVs. These two regions are hotspots of CoV phylogenetic diversity, harboring evolutionarily old and phylogenetically diverse lineages of α- and β-CoVs. South western China acted as a refugium during Quaternary glaciation for numerous plant and animal species, including several bat species, such as R. affinis [65] , Rhinolophus sinicus [66] , Myotis davidii [67] , and Cynopterus sphinx [68] . The stable and long-term persistence of bats and other mammals throughout the Quaternary may explain the deep macroevolutionary diversity of bat-CoVs in these regions [69] . Several highly significant and ancient CoV dispersal routes from these two regions have been identified in this study. Other viruses, such as the Avian Influenza A viruses H5N6, H7N9, and H5N1, also likely originated in SW and Southern Chinese regions [70] , [71] . Our findings suggest that bat host diversity is not the main driver of CoV diversity in China and that other ecological or biogeographic factors may influence this diversity. Overall, there were no significant correlations between CoV phylogenetic diversity and bat species diversity (total or sampled) for each province or biogeographic region, apart from a weak correlation between β-CoV phylogenetic diversity and the number of bat species sampled at the province level. Yet, we observed higher than expected phylogenetic diversity in several southern provinces (Hainan, Guangxi, and Hunan). These results and main conclusions are consistent and robust even when we account for geographic biases in sampling effort by analyzing random subsets of the data. Despite being an exhaustive study of bat-CoVs in China, this study had several limitations that must be taken into consideration when interpreting our results. First, only partial RdRp sequences were generated in this study and used in our phylogenetic analysis as the noninvasive samples (rectal swabs/feces) collected in this study prevented us from generating longer sequences in many cases. The RdRp gene is a suitable marker for this kind of study as it reflects vertical ancestry and is less prone to recombination than other regions of the CoV genome such as the spike protein gene [16] , [72] . While using long sequences is always preferable, our phylogenetic trees are well supported and their topology consistent with trees obtained using longer sequences or whole genomes [30] , [73] . Second, most sequences in this study were obtained by consensus PCR using primers targeting highly conserved regions. Even if this broadly reactive PCR assay designed to detect widely variant CoVs has proven its ability to detect a large diversity of CoVs in a wide diversity of bats and mammals [30] , [74] , [75] , [76] , [77] , we may not rule out that some bat-CoV variants remained undetected. Using deep sequencing techniques would allow to detect this unknown and highly divergent diversity. In this study, we identified the host taxa and geographic regions that together define hotspots of CoV phylogenetic diversity and centers of diversification in China. These findings may provide a strategy for targeted discovery of bat-borne CoVs of zoonotic or livestock infection potential, and for early detection of bat-CoV outbreaks in livestock and people, as proposed elsewhere [78] . Our results suggest that future sampling and viral discovery should target two hotspots of CoV diversification in Southern and South western China in particular, as well as neighboring countries where similar bat species live. These regions are characterized by a subtropical to tropical climate; dense, growing, and rapidly urbanizing populations of people; a high degree of poultry and livestock production; and other factors that may promote cross-species transmission and disease emergence [78] , [79] , [80] . Additionally, faster rates of evolution in the tropics have been described for other RNA viruses that could favor cross-species transmission of RNA viruses in these regions [81] . Both SARS-CoV and SADS-CoV emerged in this region, and several bat SARSr-CoVs with high zoonotic potential have recently been reported from there, although the dynamics of their circulation in wild bat populations remain poorly understood [16] , [61] . Importantly, the closest known relative of SARS-CoV-2, a SARS-related virus, was found in a Rhinolophus sp. bat in this region [20] , although it is important to note that our survey was limited to China, and that the bat hosts of this virus also occur in nearby Myanmar and Lao PDR. The significant public health and food security implications of these outbreaks reinforce the need for enhanced, targeted sampling and discovery of novel CoVs. Because intensive sampling has not, to our knowledge, been undertaken in countries bordering southern China, these surveys should be extended to include Myanmar, Lao PDR, and Vietnam, and perhaps across southeast Asia. Our finding that Rhinolophus spp. are most likely to be involved in host-switching events makes them a key target for future longitudinal surveillance programs, but surveillance targeted the genera Hipposideros and Aselliscus may also be fruitful as they share numerous β-CoVs with Rhinolophus bats. In the aftermath of the SARS-CoV and MERS-CoV outbreaks, β-CoVs have been the main focus of bat-CoV studies in China, Africa, and Europe [16] , [17] , [32] , [36] , [61] . However, we have shown that α-CoVs have a higher propensity to switch host within their natural bat reservoirs, and therefore also have a high cross-species transmission potential and risk of spillover. This is exemplified by the recent emergence of SADS-CoV in pigs in Guangdong province [17] . Two human α-CoVs, NL63 and 229E, also likely originated in bats [27] , [28] , reminding us that past spillover events from bat species can readily be established in the human population. Future work discovering and characterizing the biological properties of bat α-CoVs may therefore be of potential value for public and livestock health. Our study, and recent analysis of viral discovery rates [78] , suggests that a substantially wider sampling and discovery net will be required to capture the complete diversity of CoVs in their natural hosts and assess their potential for cross-species transmission. The bat genera Rhinolophus , Hipposideros , Myotis , and Miniopterus , all involved in numerous naturally occurring host switches throughout α-CoV evolution, should be a particular target for α-CoV discovery in China and across southeast Asia, with in vitro and experimental characterization to better understand their potential to infect people or livestock and cause disease. Bat sampling Bat oral and rectal swabs and fecal pellets were collected from 2010 to 2015 in numerous Chinese provinces (Anhui, Beijing, Guangdong, Guangxi, Guizhou, Hainan, Henan, Hubei, Hunan, Jiangxi, Macau, Shanxi, Sichuan, Yunnan, and Zhejiang). Fecal pellets were collected from tarps placed below bat colonies. Bats were captured using mist nets at their roost site or feeding areas. Each captured bat was stored into a cotton bag, all sampling was non-lethal and bats were released at the site of capture immediately after sample collection. A wing punch was also collected for barcoding purpose. Bat-handling methods were approved by Tufts University IACUC committee (proposal #G2017-32) and Wuhan Institute of Virology Chinese Academy of Sciences IACUC committee (proposal WIVA05201705). Samples were stored in viral transport medium at −80 °C directly after collection. RNA extraction and PCR screening RNA was extracted from 200 μl swab rectal samples or fecal pellets with the High Pure Viral RNA Kit (Roche) following the manufacturer’s instructions. RNA was eluted in 50 μl elution buffer and stored at −80 °C. A one-step hemi-nested reverse transcription-PCR (Invitrogen) was used to detect CoV RNA using a set of primers targeting a 440-nt fragment of the RdRp gene and optimized for bat-CoV detection (CoV-FWD3: GGTTGGGAYTAYCCHAARTGTGA; CoV-RVS3: CCATCATCASWYRAATCATCATA; CoV-FWD4/Bat: GAYTAYCCHAARTGTGAYAGAGC) [82] . For the first round PCR, the amplification was performed as follows: 50 °C for 30 min, 94 °C for 2 min, followed by 40 cycles consisting of 94 °C for 20 s, 50 °C for 30 s, 68 °C for 30 s, and a final extension step at 68 °C for 5 min. For the second round PCR, the amplification was performed as follows: 94 °C for 2 min, followed by 40 cycles consisting of 94 °C for 20 s, 59 °C for 30 s, 72 °C for 30 s, and a final extension step at 72 °C for 7 min. PCR products were gel purified and sequenced with an ABI Prism 3730 DNA analyzer (Applied Biosystems, USA). PCR products with low concentration or bad sequencing quality were cloned into pGEM-T Easy Vector (Promega) for sequencing. Positive results detected in bat genera that were not known to harbor a specific CoV lineage previously were repeated a second time (PCR + sequencing) as a confirmation. Species identifications from the field were also confirmed and re-confirmed by cytochrome (cytb) DNA barcoding using DNA extracted from the feces or swabs [83] . Only viral detection and barcoding results confirmed at least twice were included in this study. Sequence data We also added bat-CoV RdRp sequences from China available in GenBank to our dataset. All sequences for which sampling year and host or sampling location information was available either in GenBank metadata or in the original publication were included (as of March 15, 2018). Our final datasets include 630 sequences generated for this study and 616 sequences from GenBank or GISAID (list of GenBank, China National Genomics Data Center and GISAID accession numbers available in Supplementary Note 1 , and Supplementary Tables 34 , 35 , and 36 ). Nucleotide sequences were aligned using MUSCLE and trimmed to 360 base pair length to reduce the proportion of missing data in the alignments. All phylogenetic analyses were performed on both the complete data and random subset, and for α- and β-CoVs separately. Defining zoogeographic regions in China Hierachical clustering was used to define zoogeographic regions within China by clustering provinces with similar mammalian diversity [45] . Hierarchical cluster analysis classifies several objects into small groups based on similarities between them. To do this, we created a presence/absence matrix of all extant terrestrial mammals present in China using data from the IUCN spatial database [84] and generated a cluster dendrogram using the function hclust with average method of the R package stats. Hong Kong and Macau were included within the neighboring Guangdong province. We then visually identified geographically contiguous clusters of provinces for which CoV sequences are available (Fig. 1 and Supplementary Fig. 1 ). We identified six zoogeographic regions within China based on the similarity of the mammal community in these provinces: SW (Yunnan province), NO (Xizang, Gansu, Jilin, Anhui, Henan, Shandong, Shaanxi, Hebei, and Shanxi provinces and Beijing municipality), CN (Sichuan and Hubei provinces), CE (Guangxi, Guizhou, Hunan, Jiangxi, and Zhejiang provinces), SO (Guangdong and Fujian provinces, Hong Kong, Macau, and Taiwan), and HI. Hunan and Jiangxi, clustering with the SO provinces in our dendrogram, were included within the central region to create a geographically contiguous Central cluster (Supplementary Fig. 1 ). These six zoogeographic regions are very similar to the biogeographic regions traditionally recognized in China [85] . The three β-CoV sequences from HI were included in the SO region to avoid creating a cluster with a very small number of sequences. Model selection and phylogenetic analysis Bayesian phylogenetic analysis was performed in BEAST 1.8.4 [46] . Sampling years were used as tip dates. Preliminary analysis were run to select the best-fitting combination of substitution models (HKY/GTR), codon partition scheme, molecular clock (strict/lognormal uncorrelated relaxed clock), and coalescent models (constant population size/exponential growth/GMRF Bayesian Skyride). Model combinations were compared and the best-fitting model was selected using a modified Akaike information criterion implemented in Tracer 1.6 [86] . We also used TEMPEST [87] to assess the temporal structure within our α- and β-CoV datasets. TEMPEST showed that both datasets did not contain sufficient temporal information to accurately estimate substitution rates or time to the most recent common ancestor. Therefore, we used a fixed substitution rate of 1.0 for all our BEAST analysis. All subsequent BEAST analysis were performed under the best-fitting model, including an HKY substitution model with two codons partitions ((1 + 2), 3), a strict molecular clock and a constant population size coalescent model. Each analysis was run for 2.5 × 10 8 generations, with sampling every 2 × 10 4 steps. All BEAST computations were performed on the CIPRES Science Getaway Portal [88] . Convergence of the chain was assessed in Tracer so that the effective sample size (ESS) of all parameters was >200 after removing at least 10% of the chain as burn-in. Ancestral state reconstruction and transition rates A Bayesian discrete phylogeographic approach implemented in BEAST 1.8.4 was used to reconstruct the ancestral state of each node in the phylogenetic tree for three discrete traits: host family, host genus, and zoogeographic region. An asymmetric trait substitution model was applied. These analyses were performed for each trait on the complete dataset and random subsets. MCC tree annotated with discrete traits were generated in TreeAnnotator and visualized using the software SpreaD3 [89] . 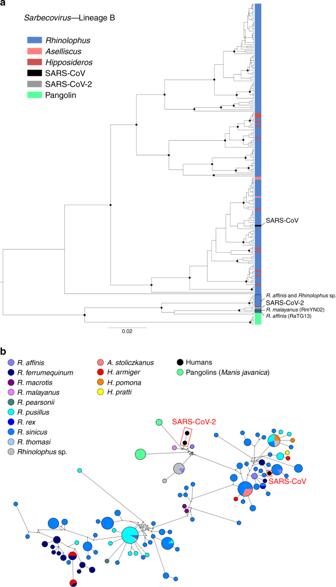For each analysis, a BSSVS was applied to estimate the significance of pairwise switches between trait states using BF as a measure of statistical significance [47] . BFs were computed in SpreaD3. BF support was interpreted according to Jeffreys in 1961 [90] (BF > 3: substantial support, BF > 10: strong support, BF > 30: very strong support, BF > 100: decisive support) and only strongly supported transitions were presented in most figures, following a strategy used in other studies [91] , [92] . We also estimated the count of state switching events (Markov jumps) [48] , [49] along the branches of the phylogenetic tree globally (for the three discrete traits) and for each strongly supported (BF > 10) transition between character states (for bat families and ecoregions only). Convergence of the MCMC runs was confirmed using Tracer. The rate of state switching events per unit of time was estimated for each CoV genus by dividing the total estimated number of state switching events by the total branch length of the MCC tree. Fig. 3: Phylogenetic relationships within theSarbecovirussubgenus (β-CoVs). Maximum clade credibility tree (a) including 202RdRpsequences from theSarbecovirussubgenus isolated in bats, two sequences of SARS-CoV-2, and one sequence of SARS-CoV isolated in humans and eight sequences isolated in Malayan pangolins (Manis javanica). Well-supported nodes (posterior probability > 0.95) are indicated with a black dot. Tip colors correspond to the host genus; SARS-CoV-2 sequences and SARS-CoV sequence are highlighted in gray and black, respectively. Median-joining network (b) including 202RdRpsequences from theSarbecoviruslineage isolated in bats, two sequences of SARS-CoV-2, and one sequence of SARS-CoV isolated in humans and eight sequences isolated in Malayan pangolins (Manis javanica). Colored circles correspond to distinct CoV sequences, and circle size is proportional to the number of identical sequences in the dataset. Small black circles represent median vectors (ancestral or unsampled intermediate sequences). Branch length is proportional to the number of mutational steps between haplotypes. To assess the phylogenetic relationships among SARS-CoV-2 and other CoVs from the Sarbecovirus subgenus, we also reconstructed an MCC tree in BEAST 1.8.4 and median‐joining network in Network 10.0 [93] , including all Sarbecovirus sequences, two sequences of SARS-CoV-2 isolated in humans (GenBank accession numbers: MN908947 and MN975262), one sequence of SARS-CoV (GenBank accession number: NC_004718), eight sequences from Malayan pangolins ( M. javanica ) (GISAID accession numbers: EPI_ISL_410538-410544, EPI_ISL_410721) and one from Rhinolophus malayanus (GISAID accession number: EPI_ISL_412977) (Supplementary Note 1 and Supplementary Table 36 ). Phylogenetic diversity The MPD and the MNTD statistics [50] and their SES were calculated for each zoogeographic region, bat family, and genus using the R package picante [94] . MPD measures the MPD among all pairs of CoVs within a host or a region. It reflects phylogenetic structuring across the whole phylogenetic tree and assesses the overall divergence of CoV lineages in a community. MNTD is the mean distance between each CoV and its nearest phylogenetic neighbor in a host or region, and therefore it reflects the phylogenetic structuring closer to the tips and shows how locally clustered taxa are. SES MPD and SES MNTD values correspond to the difference between the phylogenetic distances in the observed communities versus null communities. Low and negative SES values denote phylogenetic clustering, high and positive values indicate phylogenetic over-dispersion, while values close to 0 show random dispersion. The SES values were calculated by building null communities by randomly reshuffling tip labels 1000 times along the entire phylogeny. Phylogenetic diversity computations were performed on both the complete dataset and random subset for each trait. A linear regression analysis was performed in R to assess the correlation between CoV phylogenetic diversity (MPD) and bat species richness in China. Total species richness per province or region was estimated using data from the IUCN spatial database, while sampled species richness corresponds to the number of bat species sampled and tested for CoV per province or region in our datasets. The inter-region and inter-host values of MPD (equivalent to phylogenetic β diversity), corresponding to the MPD among all pairs of CoVs from two distinct hosts or regions, and their SES were estimated using the function comdist of the R package phylocomr [95] . The matrices of inter-region and inter-host MPD were used to cluster zoogeographic regions and bat hosts in a dendrogram according to their evolutionary similarity (phylo-ordination) using the function hclust with complete linkage method of the R package stats (R core team). These computations were performed on both the complete dataset and random subset. Mantel tests and isolation by distance Mantel tests performed in ARLEQUIN 3.5 [96] were used to compare the matrix of viral genetic differentiation ( F ST ) to matrices of host phylogenetic distance and geographic distance in order to evaluate the role of geographic isolation and host phylogeny in shaping CoV population structure. The correlation between these matrices was assessed using 10,000 permutations. To gain more resolution into the process of evolutionary diversification, these analyses were also performed at the host genus and province levels. To calculate phylogenetic distances among bat genera, we reconstructed a phylogenetic tree, including a single sequence for all bat species included in our dataset. Pairwise patristic distances among tips were computed using the function distTips in the R package adephylo [97] . We then averaged all distances across genera to create a matrix of pairwise distances among bat genera. Pairwise Euclidian distances were measured between province centroids and log transformed. Mantel tests were performed with and without genera and provinces, including <4 viral sequences to assess the impact of low sample size on our results. Reporting summary Further information on research design is available in the Nature Research Reporting Summary linked to this article.